A two-dimensional spin liquid in quantum kagome ice Actively sought since the turn of the century, two-dimensional quantum spin liquids (QSLs) are exotic phases of matter where magnetic moments remain disordered even at zero temperature. Despite ongoing searches, QSLs remain elusive, due to a lack of concrete knowledge of the microscopic mechanisms that inhibit magnetic order in materials. Here we study a model for a broad class of frustrated magnetic rare-earth pyrochlore materials called quantum spin ices. When subject to an external magnetic field along the [111] crystallographic direction, the resulting interactions contain a mix of geometric frustration and quantum fluctuations in decoupled two-dimensional kagome planes. Using quantum Monte Carlo simulations, we identify a set of interactions sufficient to promote a groundstate with no magnetic long-range order, and a gap to excitations, consistent with a Z 2 spin liquid phase. This suggests an experimental procedure to search for two-dimensional QSLs within a class of pyrochlore quantum spin ice materials. In a two-dimensional (2D) quantum spin liquid (QSL) state, strong quantum fluctuations prevent the ordering of magnetic spins, even at zero temperature. The resulting disordered phase can potentially be a remarkable state of matter, supporting a range of exotic quantum phenomena. Some, such as emergent gauge structures and fractional charges, are implicated in a wide range of future technologies like high-temperature superconductivity [1] , [2] and topological quantum computing [3] . It is therefore remarkable that, despite extensive examination of the basic theoretical ingredients required to promote a 2D QSL in microscopic models [4] , [5] , the state remains elusive, with only a few experimental candidates existing today [6] , [7] . Recently, the search for QSL states has turned to consider quantum fluctuations in the so-called spin ice compounds [8] . In these systems, magnetic ions reside on a pyrochlore lattice—a non-Bravais lattice consisting of corner-sharing tetrahedra. Classical magnetic moments (described by Ising spins) on the pyrochlore lattice can be geometrically frustrated at low temperatures, leading to spin configurations that obey the so-called ‘ice rules’, a mapping to the proton-disorder problem in water ice [9] . The ice rules result in a large set of degenerate ground states—a classical spin liquid with a finite thermodynamic entropy per spin [10] , [11] . Two canonical materials, Ho 2 TiO 7 and Dy 2 Ti 2 O 7 , have been demonstrated to manifest spin ice behaviour, and experiments and theory enjoy a healthy dialogue due to the existence of classical microscopic models capable of describing a wide range of experimental phenomena [10] . Classical spin ice pyrochlores are conjectured to lead to QSLs in the presence of the inevitable quantum fluctuations at low temperatures [4] , [8] . The effects of certain types of quantum fluctuations on the spin ice state have been investigated theoretically [12] and numerically [13] , [14] , where they have been demonstrated to lift the classical degeneracy and promote a three-dimensional (3D) QSL phase with low-energy gapless excitations that behave like photons [12] , [13] . In several related pyrochlore compounds, particularly Tb 2 Ti 2 O 7 , Yb 2 Ti 2 O 7 , Pr 2 Zr 2 O 7 and Pr 2 Sn 2 O 7 , quantum effects have been observed, which make them natural candidates to search for such 3D QSLs [15] , [16] , [17] . In an attempt to elucidate the microscopic underpinnings of these and related materials, recent theoretical studies have produced a general low-energy effective spin-1/2 model for magnetism in rare earth pyrochlores [18] , [19] , [20] . In an important development, Huang, Chen and Hermele [21] have shown that, on the pyrochlore lattice, strong spin-orbit coupling can lead to Kramers doublets with dipolar-octupolar character in d - and f -electron systems. This allows for a specialization of the general effective model to one without the debilitating ‘sign problem’—amenable to solution through quantum Monte Carlo (QMC) methods—thus admitting a systematic search for QSL phases via large-scale computer simulations. Using large-scale QMC simulations, we show that a two-dimensional model on the kagome lattice descending from the quantum Hamiltonian discussed by Huang, Chen and Hermele [21] exhibits an exotic disordered phase—a quantum kagome ice state—in a wide range of Hamiltonian parameters. Such a state displays exponentially decaying correlations and is consistent with a gapped QSL phase. These results suggest an alternative experimental route to search for the long-sought QSL phase in two dimensions starting from quantum spin ice pyrochlore materials subject to an external field along the [111] direction. A quantum kagome ice model While the possibility for 3D QSLs in the above compounds is intriguing, spin ice materials offer a compelling mechanism for dimensional reduction to 2D, since single-ion anisotropy constrains magnetic moments to point along the local tetrahedral symmetry axes in the pyrochlore lattice. This mechanism consists of the application of an external magnetic field along the global [111] crystallographic direction that partially lifts the spin ice degeneracy by pinning one spin per tetrahedron. As illustrated in Fig. 1a , this [111] magnetic field effectively decouples spins between the alternating kagome and triangular layers of the original pyrochlore structure. To simplest approximation, the system becomes a two-dimensional system of stacked kagome planes [22] , [23] , [24] , [25] , where spins on the intervening triangular planes align in the direction of the field (becoming energetically removed from the problem), while those in the kagome plane ( Fig. 1b ) remain partially disordered. These kagome spins retain a fraction of the zero-field spin ice entropy, though still preserving the spin ice rules (two-in, two-out) of the parent pyrochlore system. This leads to classically disordered state, termed kagome ice [22] , [24] , [25] , [26] , evidenced to date in several experimental studies on spin ice materials [27] , [28] , [29] . 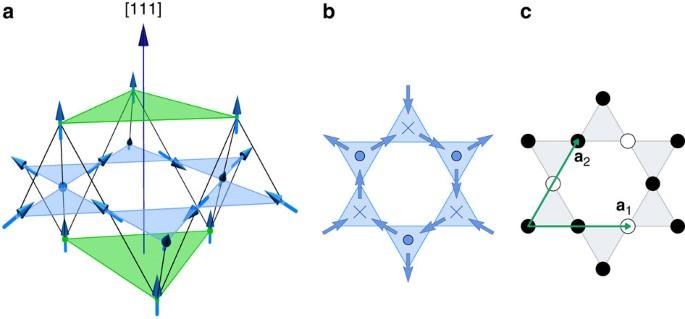Figure 1: From pyrochlore spin ice to kagome ice. (a) The pyrochlore lattice viewed as a set of alternating kagome (blue) and triangular (green) layers along the [111] direction. Spins on the pyrochlore lattice (blue arrows) satisfy the ‘ice rules’: two-in, two-out of each tetrahedron. (b) Two-dimensional projection of the pyrochlore spin configuration onto a kagome plane (blue arrows). At the centre of each triangle is a representation of the out-of-plane spin: dots (crosses) refer to a spin pointing inwards (outwards) of each tetrahedron ina. (c) The associated pseudo-spinconfiguration where filled (empty) circles represents a pseudo-spin up (down). Our quantum Monte Carlo simulations of the pseudo-spin Hamiltonian are defined on periodic tori spanned by the primitive vectorsa1anda2, where‖a1‖=‖a2‖=2. Figure 1: From pyrochlore spin ice to kagome ice. ( a ) The pyrochlore lattice viewed as a set of alternating kagome (blue) and triangular (green) layers along the [111] direction. Spins on the pyrochlore lattice (blue arrows) satisfy the ‘ice rules’: two-in, two-out of each tetrahedron. ( b ) Two-dimensional projection of the pyrochlore spin configuration onto a kagome plane (blue arrows). At the centre of each triangle is a representation of the out-of-plane spin: dots (crosses) refer to a spin pointing inwards (outwards) of each tetrahedron in a . ( c ) The associated pseudo-spin configuration where filled (empty) circles represents a pseudo-spin up (down). Our quantum Monte Carlo simulations of the pseudo-spin Hamiltonian are defined on periodic tori spanned by the primitive vectors a 1 and a 2 , where ‖ a 1 ‖ = ‖ a 2 ‖ =2. Full size image The above observations lead to a natural microscopic mechanism to search for 2D QSL behaviour [30] . First, one begins with classical nearest-neighbour spin ice in an applied [111] field, so as to promote the aforementioned kagome ice state. This model maps to a projected pseudo-spin Ising model with a symmetry-breaking Zeeman field h , arising from a combination of the physical [111] field and the original pyrochlore spin exchange interaction ( Fig. 1c ). For moderate h , the classical ground state retains an extensive degeneracy, before becoming a fully polarized ferromagnetic state for h / J z >2. Next, to include the effect of quantum fluctuations, one may add exchanges from the recent quantum spin ice models [18] , [19] , [20] , [21] . We consider only those quantum fluctuations discussed by Huang et al. [21] , to obtain a pseudo-spin Hamiltonian on the kagome lattice, Here, S r are spin-1/2 operators, with a global z axis ( and in Fig. 1c ). This Hamiltonian cannot be solved exactly by analytical techniques; however large-scale QMC simulations are possible in a parameter regime ( J ± ≥0) devoid of the prohibitive sign problem. One can imagine a 2D QSL state arising conceptually by considering the quantum fluctuations J ± and J ±± as perturbations on the classical kagome ice limit, where only diagonal terms J z >0 and are present. Previously, large-scale QMC simulations have been performed on the kagome model in the limit J ± >0 and J ±± =0 (refs 31 , 32 ) (a parameter regime where the Hamiltonian retains U(1) invariance). In that case, quantum fluctuations promote an in-plane ferromagnetic (FM) phase for h =0, and a valence bond-solid (VBS—a conventional symmetry broken phase) for h >0. Thus, it happens that fluctuations of the form induced by J ± are not sufficient to promote a 2D QSL state. However, there remains the theoretical possibility of a gapped Z 2 QSL phase promoted by the J ±± quantum fluctuations. As detailed in the Supplementary Note 1 and Supplementary Fig. 1 , the local constraints of classical kagome ice can be translated into a charge-free condition on the dual honeycomb lattice. Then, the full Hamiltonian (1) can be re-cast as a system of interacting bosonic spinons coupled to a compact U(1) gauge field on the dual lattice. In the limit of J ± =0, this theory is expected to exhibit two distinct phases. One is a confined phase, corresponding to a conventional spin-ordered state; the other is a deconfined Z 2 QSL phase [20] , [21] , [33] . From these simple arguments it is conceivable that these two phases exist in the phase diagram of equation (1). In the next section, we set J ± =0 and explore this possibility for all parameter regimes J ±± / J z and h / J z , using non-perturbative, unbiased QMC simulations. Before proceeding with the description of the QMC results, we emphasize that neither our simulations nor the analysis of the resulting lattice gauge theory are restricted to states within the ice manifold. Quantum Monte Carlo results We implement a finite-temperature Stochastic Series Expansion [34] , [35] , [36] (SSE) QMC algorithm with directed loop updates in a 2+1 dimensional simulation cell, designed specifically to study the Hamiltonian equation (1) with J ± =0 (for details, see the Methods Summary). Note, this Hamiltonian explicitly breaks U(1) invariance, retaining global Z 2 symmetries. By a canonical transformation, S ± →± iS ± ; we simulate only J ±± <0, without loss of generality [21] . Various measurements are possible in this type of QMC simulation. Simplest are the standard SSE estimators for energy, magnetization , and uniform spin susceptibility . The latter two allow us to map out the broad features of the phase diagram. Further, we measure the off-diagonal spin structure factor [37] Here, r i points to the sites of the underlying triangular lattice (containing N s sites) of the kagome lattice (containing V =3 × N s sites). The vectors α are the position of each site within the unit cell with respect to the vector r i . This quantity allows us to define, for this spin Hamiltonian, the analogue of a condensate fraction in bosonic systems [38] , [39] , which detects transverse magnetic ordering. We define as the ratio of largest eigenvalue n M of the one-body density matrix to the number of sites V . The eigenvalues of ρ i , j coincide with for a translationally invariant system. 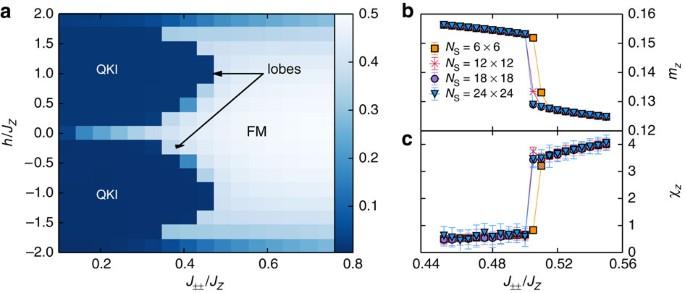Figure 2: Phase diagram of the model. (a) Phases of the two-dimensional quantum kagome ice model forJ±=0 as a function ofh/JzandJ±±/Jz. The colour scale represents the zero-momentum occupationf0obtained from aNs= 6 × 6 lattice and temperatureT=Jz/24. In the quantum kagome ice lobes (QKI),and, whereas in the ferromagnetic (FM) phase. Magnetization (b) and uniform susceptibility (c) as a function ofJ±±/Jzentering the candidateZ2quantum spin liquid lobe at fixedh/Jz=0.833.Ns=6 × 6, 12 × 12, 18 × 18 and 24 × 24 are represented by orange squares, red crosses, purple circles and blue down triangles, respectively. Solid lines are guides to the eye. The error bars represent the one s.d. statistical uncertainty. Note that a fully spin-polarized phase occurs forh/Jz≥2, which is not illustrated in this phase diagram. Figure 2a shows the QMC phase diagram for the J ± =0 model of equation (1), using data for the condensate fraction f 0 . Careful finite-temperature and finite-size scaling, performed up to lattice sizes of V = L × L × 3=39 × 39 × 3 and β = J z / T =96, is detailed in the Supplementary Information ( Supplementary Figs 2 and 3 and Supplementary Note 2 ). The magnetization curve and the uniform spin susceptibility across the phase boundary at fixed h / J z =0.833 are presented in Fig. 2a,b . The data clearly indicate the existence of two magnetized lobes on the phase diagram for J ±± / J z <0.5 and h / J z ≠0, where the zero-momentum condensate fraction of a surrounding FM phase is destroyed by a phase transition (which appears to be first order). The lobes have magnetizations of m ≈−1/6 and m ≈+1/6 for h / J z <0 and h / J z >0, respectively. The FM phase has a finite uniform susceptibility χ z , while the lobe phases retain a small but finite χ z that can be understood by the nature of the quantum fluctuation as a spin pair interaction, which does not conserve the total magnetization . As discussed above, the phase in these lobes is a candidate for supporting a 2D QSL state. Figure 2: Phase diagram of the model. ( a ) Phases of the two-dimensional quantum kagome ice model for J ± =0 as a function of h / J z and J ±± / J z . The colour scale represents the zero-momentum occupation f 0 obtained from a N s = 6 × 6 lattice and temperature T = J z /24. In the quantum kagome ice lobes (QKI), and , whereas in the ferromagnetic (FM) phase . Magnetization ( b ) and uniform susceptibility ( c ) as a function of J ±± / J z entering the candidate Z 2 quantum spin liquid lobe at fixed h / J z =0.833. N s =6 × 6, 12 × 12, 18 × 18 and 24 × 24 are represented by orange squares, red crosses, purple circles and blue down triangles, respectively. Solid lines are guides to the eye. The error bars represent the one s.d. statistical uncertainty. Note that a fully spin-polarized phase occurs for h / J z ≥2, which is not illustrated in this phase diagram. Full size image To examine this hypothesis, we perform a detailed search for ordered structures in the lobes. In related models, particularly the spin-1/2 XXZ model on kagome (that is, J ±± =0 and J ± >0) [31] , [32] , the analogous lobes support a conventional VBS phase, which is evident in the diagonal structure factor: , where If there is long-range order then will scale with system size for at least one value of q . We also measure the bond-bond structure factor using a four-point correlation function. where . Nearest neighbour sites i aα and j aα belong to bond α in a unit cell located at position r a . Again, if there is pair long-range order then should scale with system size for at least one value of q , with which we define B q = BB q / V . 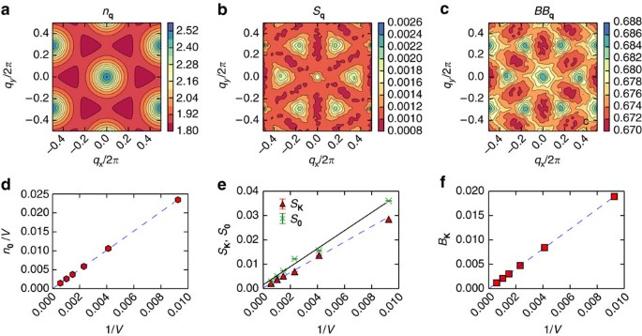Figure 3: Structure factors and absence of order in the lobe. Off-diagonalnq(a), diagonalSq(b), and bondBBq(c) structure factors inside the lobe for a system withNs=24 × 24,h/Jz=0.8333,J±±/Jz=0.495 andT=Jz/48. In each panel, the colour scale represents the intensity of the structure factor. The corresponding finite-size scaling of candidate peaks atqvalues where local maxima occur in the structure factorsn0(d)(red hexagons),S0andSK(e)(red triangles and green, respectively), andBK(f)(red squares). The error bars represent the one s.d. statistical uncertainty. Linear fits to the data in panels (d–f) are represented as blue dashed and black solid lines. The zero-momentum peak ofBB0in panel (c) has been removed. In each panel, the colour scales represent the intensity of the structure factor. Figure 3 illustrates the various q -dependent structure factors for spin and bond order. These structure factors display diffuse peaks at various wave vectors, notably q = 0 , q = K =(2 π /3,0), and symmetry-related momenta. Such peaks would indicate the presence of long-range order, should they sharpen, and survive in intensity in the infinite-size limit, where S / V would correspond to an order parameter squared. In Fig. 3d through Fig. 3f , we examine this through a standard finite-size scaling analysis, for several candidate peaks for each of the structure factors. Further scaling analysis, including larger system sizes, is presented and analysed in the light of perturbative arguments in the Supplementary Information ( Supplementary Note 3 and Supplementary Figs 2 and 4 ). In each case, the QMC data indicates a scaling of each order parameter to zero in the limit V →∞. Note in particular, the largest value of B q corresponds to q = 0 , which remains finite as V →∞, meaning that the bond expectation values is finite in the lobes. This is expected as represents the kinetic energy of quantum fluctuations in the system, and thus it should be finite in all phases. More importantly, the data indicate that in the limit of V →∞ this quantity is the same on all bonds of the unit cell of the kagome lattice, meaning that there is no breaking of space-group symmetry (see Supplementary Note 4 and Supplementary Figs 5–7 ). Figure 3: Structure factors and absence of order in the lobe. Off-diagonal n q ( a ), diagonal S q ( b ), and bond BB q ( c ) structure factors inside the lobe for a system with N s =24 × 24, h / J z =0.8333, J ±± / J z =0.495 and T = J z /48. In each panel, the colour scale represents the intensity of the structure factor. The corresponding finite-size scaling of candidate peaks at q values where local maxima occur in the structure factors n 0 ( d )(red hexagons), S 0 and S K ( e )(red triangles and green, respectively), and B K ( f )(red squares). The error bars represent the one s.d. statistical uncertainty. Linear fits to the data in panels ( d – f ) are represented as blue dashed and black solid lines. The zero-momentum peak of BB 0 in panel ( c ) has been removed. In each panel, the colour scales represent the intensity of the structure factor. Full size image Finally, as the above data suggest the existence of a phase that is homogeneous, disordered and quantum-mechanically fluctuating at extremely low temperatures, one should also examine whether the energy for excitations out of this ground state is gapped or gapless. Although a direct measurement of the gap is not possible in this type of SSE QMC method, we can indirectly probe its existence by looking at the decay of real-space correlations. In Fig. 4 , we compare the decay of single-particle correlations between the m z =±1/6 magnetization lobes and the adjacent FM ordered phase. For the system size studied, it is clear that correlations in the lobe are consistent with exponential decay, and therefore indicative of a gap. In contrast, in the FM phase the correlations quickly reach a finite value, indicating symmetry breaking (additional details about the nature the FM phase are discussed in Supplementary Figs 8–10 and Supplementary Note 5 ). Similarly, the diagonal part of the spin correlation function is consistent with exponential decay both in the lobes and in the FM phase (not illustrated). 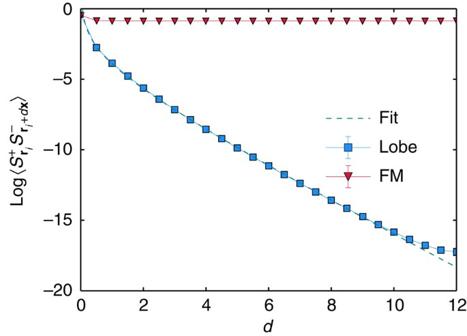Figure 4: Exponential decay of correlation functions. The off-diagonal spin correlation function as a function of distance along thexdirection for a system withNs=24 × 24 andT=Jz/48 in the candidate spin liquid phase (blue squares) and in the ferromagnet (FM)(red triangles). The dashed line corresponds to a fit of the numerical data to the function. The error bars represent the one s.d. statistical uncertainty. Figure 4: Exponential decay of correlation functions. The off-diagonal spin correlation function as a function of distance along the x direction for a system with N s =24 × 24 and T = J z /48 in the candidate spin liquid phase (blue squares) and in the ferromagnet (FM)(red triangles). The dashed line corresponds to a fit of the numerical data to the function . The error bars represent the one s.d. statistical uncertainty. Full size image Thus, our QMC results have elucidated a phase diagram for our kagome pseudo-spin XYZ model (with J ± =0), which contains a predominant FM phase, surrounding lobes of an exotic disordered m z =±1/6 magnetization phase. As our dual gauge theory (detailed in the Supplementary Note 1 ) indicates that these lobes may realize a QSL with an emergent Z 2 gauge symmetry, it is clear that further simulation work should be carried out to address this hypothesis. To confirm the presence of a Z 2 QSL, one requires evidence of either excitations consistent with this gauge structure (for example, magnetic spinons or non-magnetic visons at non-zero temperature) or a smoking gun such as the topological entanglement entropy [40] , [41] . Such evidence, although demonstrated in the past with SSE QMC [42] , [43] , is resource-intensive to obtain, requiring high numerical precision at very low temperatures, and thus outside of the scope of the present manuscript. However, we also note that, due to the presence of only a discrete symmetry in our kagome XYZ model, an emergent Z 2 structure is not strictly required by the Lieb-Schultz-Mattis-Hastings (LSMH) theorem [44] , [45] , [46] , which states that a system with half-odd-integer spin in the unit cell cannot have a gap and a unique ground state. In higher-symmetry Hamiltonians, the requirements of the LSMH theorem are satisfied in a gapped QSL phase by the topological degeneracy, which is a consequence of the emergent discrete gauge symmetry. For our Hamiltonian with a gapped QSL arising in a model with only global discrete symmetries, an emergent gauge structure is not required. Rather, it is possible that the groundstate is a quantum paramagnet. In contrast, other types of emergent gauge structure, topological order or other exotic phenomena are theoretically possible. Fortunately, the nature of this Hamiltonian, which is among the first to show a 2D QSL phase with only nearest-neighbour interactions, lends itself exceedingly well to study by sign-problem-free QMC simulations. We therefore expect a large number of studies in the near future will help elucidate the precise nature of this QSL phase. Through extensive quantum Monte Carlo simulations, we have studied a sign-problem-free model of frustrated quantum spins interacting on a two-dimensional kagome lattice. This model is descendent from a more general quantum XYZ Hamiltonian discussed by Huang, Chen and Hermele [21] , derived for the three-dimensional pyrochlore lattice, when subject to a magnetic field along the [111] crystallographic direction. For a large range of Hamiltonian parameters, the QMC data uncover an exotic disordered phase that breaks no symmetries, has strong quantum mechanical fluctuations and exponentially decaying correlations—a candidate gapped QSL phase. This discovery is consistent with an analytical dual gauge theory (detailed in the Supplementary Note 1 ), which indicates that, in the limit of small quantum fluctuations, the phase could be a 2D QSL with an emergent Z 2 gauge symmetry. Our work suggests a new experimental avenue to search for the highly coveted QSL phase in two dimensions. Previous efforts have focused largely on SU(2) Hamiltonians on kagome or triangular lattice materials [6] , [7] . In contrast, we propose to concentrate the search on the quantum spin ice pyrochlore materials, subject to an external field along the [111] direction. Such kagome ice phases have been identified in various materials in the past. A closer look at several quantum spin ice candidates is warranted, particularly in materials where strong quantum fluctuations are known to exist, such as Tb 2 Ti 2 O 7 , Yb 2 Ti 2 O 7 , Pr 2 Zr 2 O 7 and Pr 2 Sn 2 O 7 . While Hamiltonians describing some of these materials may include additional interactions [18] not considered in equation (1), our study highlights the importance of the of J ±± term, which is present for instance in Yb 2 Ti 2 O 7 (ref. 47 ), and promotes spinon pairing required in the formation of a Z 2 spin liquid. As the phase found in this study has a gap, it is necessarily protected against any local perturbation as long as the effective energy scale of the perturbation is smaller than the gap, and thus it may still be realized even in the presence of additional perturbations. Other candidate materials where the Hamiltonian in equation (1) may be explicitly relevant include Nd 2 B 2 O 7 (where B=Zr and Sn), rare earth spinels like CdEr 2 Se 4 , and Dy pyrochlores, though in the latter the effect of dipolar interactions need be considered [21] . In light of recent experiments [48] that suggest the oft-studied classical spin ice state is only metastable in Dy 2 Ti 2 O 7 , it would seem prudent to re-examine the kagome ice state of this material using similar long-timescale techniques, to ascertain whether evidence of a QSL state may be present yet dynamically inhibited in the short-timescale studies performed to date. Finally, we note that recent work by Glaetzle et al. have demonstrated that precisely our Hamiltonian (equation (1)) can be realized experimentally with cold alkali atoms stored in optical or magnetic trap arrays [49] . Such a proposal suggests that Quantum Kagome Ice may actually be realized in engineered systems of laser-dressed Rydberg atoms in the very near future. Computational details We developed a Stochastic Series Expansion [34] (SSE) QMC algorithm in the global S z basis designed to study the Hamiltonian equation (1) with J ± =0 at finite temperature, using a 2+1-dimensional simulation cell. Within the SSE, the Hamiltonian was implemented with a triangular plaquette breakup [36] , which helps ergodicity in the regime where J z / J ±± is large. Using this Hamiltonian breakup, the standard SSE-directed loop equations [35] were modified to include sampling of off-diagonal operators of the type . The resulting algorithm is highly efficient, scaling linearly in the number of lattice sites V and the inverse temperature β . This scaling is modified to V 2 β in the cases where a full q -dependent structure factor measurement is required. The program was implemented in Fortran and verified by comparing results for small clusters with exact diagonalization data (See Supplementary Fig. 11 for an energy comparisons with ED and temperature convergence of the energy for larger system sizes). For each set of parameters in equation (1), the simulation typically requires 10 7 QMC steps, with ∼ 10% additional equilibration steps. The data presented in this paper required computational resources equivalent to 155 CPU core-years, run on a high-performance computing (HPC) cluster with Intel Xeon CPUs running at 2.83 GHz clock speed. How to cite this article: Carrasquilla, J. et al. A two-dimensional spin liquid in quantum kagome ice. Nat. Commun. 6:7421 doi: 10.1038/ncomms8421 (2015).